Adipocytes arise from multiple lineages that are heterogeneously and dynamically distributed Adipose tissue development is poorly understood. Here we use a lineage-tracing strategy optimal for adipocytes to provide evidence that Myf5 precursors are not the exclusive source of brown adipocytes and contribute more to the mature white and brite adipocyte populations than previously thought. Moreover, Myf5-lineage distribution in adipose tissue changes in response to modifiable and non-modifiable factors. We also find that the Pax3 lineage largely overlaps with the Myf5 lineage in brown fat and subcutaneous white fat, but exhibits gender-linked divergence in visceral white fat while the MyoD1 lineage does not give rise to any adipocytes. Finally, by deleting insulin receptor beta in the Myf5 lineage, we provide in vivo evidence that the insulin receptor is essential for adipogenesis and that adipocyte lineages have plasticity. These data establish a conceptual framework for adipose tissue development and could explain body fat patterning variations in healthy and lipodystrophic or obese humans. Adipose tissue development is not well understood. One view is that adipose tissue is a single organ that develops from a single lineage [1] , [2] , [3] , [4] . However, lipodystrophies often manifest as lipid distribution disorders in which regionalized depot atrophy coexists with preservation and often expansion of other depots [5] . The basis for this regionalization is not understood. Adipose tissues exist in multiple discrete white (WAT) and brown (BAT) depots. WAT is typically generalized as being subcutaneous or visceral [2] , [6] . Visceral WAT is considered unfavourable because its accumulation (for example, in obesity) correlates with metabolic disease, while subcutaneous WAT is considered more metabolically favourable because its accumulation can be protective, although this generalization is likely oversimplified because metabolic properties vary between visceral depots and even between adipocytes within the same depot [2] , [6] . Why this metabolic heterogeneity exists within and between depots is also not understood. One possible explanation is that adipocytes arise from diverse lineages and that this influences fat distribution and function. However, the ability to determine this is precluded by the fact that the developmental origin of adipocytes is largely unknown [7] . We recently provided both genetic and lineage-tracing evidence that brown adipocytes and a subset of white adipocytes descend from progenitors that express Myf5 (that is, myf5-cre ), which may originate in the dermomyotome [8] , [9] , and were previously thought to give rise to brown adipocytes and myocytes, but not to any white adipocyte [10] . However, owing to inefficiencies associated with using cytoplasmic reporters (for example, R26R-LacZ ; R26R-YFP ) in lipid-laden adipocytes, our previous ability to accurately quantify the Myf5-lineage contribution to each depot in vivo was limited to the precursor pool and the number of mature adipocytes traced with Myf5-Cre could not be determined [8] . Myf5 along with Pax3 and MyoD1 are transcription factors that function in a classic myogenic transcriptional cascade [9] . During embryonic muscle development, Myf5 is thought to function downstream or simultaneously with Pax3 and upstream of MyoD1, but whether Pax3- and/or MyoD1-expressing precursors also give rise to brown or white adipocytes in vivo is not known. Here, by lineage tracing we quantify the Myf5-lineage contribution to the mature brown and white adipocyte population by combining a Myf5-Cre knockin allele with a reporter optimal for fluorescently labelling mature adipocytes. By a similar strategy, we also trace the fate in adipose tissue of precursors that express Pax3-Cre and MyoD1-Cre. We find that the Myf5-Cre and Pax3-Cre adipose tissue lineages largely overlap, but also exhibit some significant differences, while MyoD1-Cre does not label any adipocytes. We additionally uncover evidence of lineage dynamics and plasticity. These results help clarify the Myf5-lineage contribution to adipose tissue and provide support for a model in which brown, white and brite adipocytes have multiple developmental origins. Strategy for tracing adipocyte lineages We recently discovered in a conditional gene-knockout study combined with lineage tracing that Myf5-Cre targets a subset of white adipocytes in addition to brown adipocytes [8] . However, at that time were using cytoplasmic reporters for lineage tracing (that is, R26R-YFP and R26R-LacZ ) on fixed tissues and because white adipocytes are filled with lipid and contain very little cytoplasm, we could not reliably determine how many mature adipocytes were actually traced with Myf5-Cre. To overcome this roadblock, we switched to the R26R-mTmG reporter for lineage tracing, which is a dual-colour labelling system that utilizes membrane-targeted fluorescent reporters [11] . The use of membrane-targeted reporters alleviates the caveat of using cytoplasmic reporters in adipocytes and allows fluorescence detection at single-cell resolution in whole-mount preparations. In Cre-expressing mice that harbour the R26R-mTmG reporter, all Cre + cells and their descendants are irreversibly labelled with membrane-targeted green fluorescent protein (mGFP) while all Cre neg lineages express membrane-targeted Tomato fluorescent protein (mTFP). As a positive control we generated adiponectin-cre;mTmG mice in which only mature adipocytes are labelled mGFP + ( Supplementary Fig. 1a ); as a negative control we analysed R26R-mTmG mice in which all cells are mTFP + ( Supplementary Fig. 1b ). To compare the Myf5, Pax3 and MyoD lineage contributions globally to adipose tissue, we generated myf5-cre;mTmG , pax3-cre;mTmG and MyoD1-cre;mTmG mice by combining the R26R-mTmG reporter with Myf5-Cre, Pax3-Cre and MyoD1-Cre knockin alleles [12] , [13] , [14] in C57Bl/6J mice ( Fig. 1a ). Notably, while mGFP + expression in the strictest sense only indicates that the endogenous promoter is or was previously active in the cell lineage, we refer here to labelled cells as being Myf5-lin +/neg , Pax3-lin +/neg or MyoD-lin +/neg , respectively. We determined that skeletal muscles (quadriceps, gastrocnemius, triceps and trapezius) are uniformly mGFP + in the myf5-cre;mTmG , pax3-cre;mTmG and myoD1-cre;mTmG mice, while the liver in each strain is mTFP + ( Supplementary Fig. 2a,b ). Having validated the robustness of the reporter and functionality of each Cre driver, we proceeded to use the myf5-cre;mTmG , pax3-cre;mTmG and MyoD1-cre;mTmG mice to perform lineage tracing of all major adipose tissue depots ( Fig. 1b ). 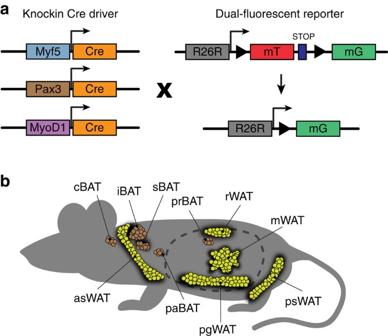Figure 1: Lineage-tracing strategy. (a) Cre drivers and fluorescent reporter system used in this study. Each Cre driver is a knockin allele meaning Cre activity is indicative of the activity of the endogenous promoter. (b) Anatomical disposition of BAT and WAT depots examined in this study. Interscapular BAT (iBAT), subscapular BAT (sBAT), cervical BAT (cBAT), peri-aortic BAT (paBAT), peri-renal BAT (prBAT), anterior-subcutaneous WAT (asWAT), posterior-subcutaneous WAT (psWAT), retroperitoneal WAT (rWAT), perigonadal WAT (pgWAT) and mesenteric WAT (mWAT) depots are indicated. Figure 1: Lineage-tracing strategy. ( a ) Cre drivers and fluorescent reporter system used in this study. Each Cre driver is a knockin allele meaning Cre activity is indicative of the activity of the endogenous promoter. ( b ) Anatomical disposition of BAT and WAT depots examined in this study. Interscapular BAT (iBAT), subscapular BAT (sBAT), cervical BAT (cBAT), peri-aortic BAT (paBAT), peri-renal BAT (prBAT), anterior-subcutaneous WAT (asWAT), posterior-subcutaneous WAT (psWAT), retroperitoneal WAT (rWAT), perigonadal WAT (pgWAT) and mesenteric WAT (mWAT) depots are indicated. Full size image Myf5-Cre and Pax3-Cre mark similar adipocyte populations First, we asked whether Pax3-Cre and/or MyoD1-Cre trace adipocyte precursor cells (APCs) in patterns similar to Myf5-Cre. Importantly, the percentages of Myf5-lin + (that is, mGFP + ) APCs in each depot match our previous data obtained with the cytoplasmic R26R-YFP reporter ( Fig. 2a ) [8] , confirming the R26R-mTmG reporter’s accuracy. Pax3-Cre lineage tracing recapitulates a nearly identical pattern to that of the Myf5-Cre in the APC populations except for one major depot difference: 31.2% of the APCs in male perigonadal WAT (pgWAT) are Pax3-lin + compared with only 2.6% being Myf5-lin + ( Fig. 2a,b ). In contrast, <1% of the female pgWAT APCs are Pax3-lin + hinting at a gender-linked difference in Pax3-lineage distribution ( Fig. 2b ). The MyoD1-Cre does not label APCs in any depot we examined ( Fig. 2c ) suggesting that developmental lineages expressing MyoD1 do not typically give rise to adipocytes. We conclude that Myf5-Cre and Pax3-Cre label similar pools of APCs in most depots with the one exception being male pgWAT, in which Pax3-Cre but not Myf5-Cre labels a significant number of APCs. 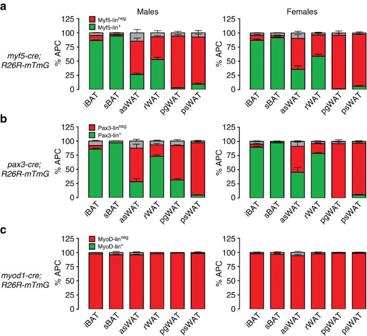Figure 2: Lineage-tracing of adipocyte precursor cells (APCs). (a–c) Number of mTFP+and mGFP+APCs isolated from each of the indicated depots from 6-week-oldmyf5-cre;R26R-mTmG(a),pax3-cre;R26R-mTmG(b) andmyod1-cre;R26R-mTmGmice (c). Data from males and females are shown separately (n=3–5; mean+s.e.m.). A small number of cells in each case that could not be distinguished are indicated in grey. Figure 2: Lineage-tracing of adipocyte precursor cells (APCs). ( a – c ) Number of mTFP + and mGFP + APCs isolated from each of the indicated depots from 6-week-old myf5-cre;R26R-mTmG ( a ), pax3-cre;R26R-mTmG ( b ) and myod1-cre;R26R-mTmG mice ( c ). Data from males and females are shown separately ( n =3–5; mean+s.e.m.). A small number of cells in each case that could not be distinguished are indicated in grey. Full size image Brown adipocytes have multiple origins Next, we asked whether all mature brown adipocytes arise from Myf5-Cre-expressing precursors as one model posits [15] . In the interscapular and subscapular depots (iBAT and sBAT), we find that 99% and 100% of the brown adipocytes, respectively, are indeed Myf5-lin + in both males and females ( Fig. 3a ; Supplementary Fig. 3a ). However, in cervical BAT (cBAT) only 58% of male and 66% of female brown adipocytes are traced with Myf5-Cre exhibiting a mosaic distribution pattern ( Fig. 3a ; Supplementary Fig. 3a ). In peri-renal BAT and peri-aortic (paBAT) brown fat, no brown adipocytes are Myf5-lin + ( Fig. 3a ; Supplementary Fig. 3a ). We confirmed the brown fat identity of each individual depot by showing high levels of ucp1 , prdm16 and cidea messenger RNA expression compared with WATs, by haematoxylin and eosin staining showing multilocular lipid droplets, and by UCP1 immunohistochemistry ( Supplementary Fig. 4 ). These results indicate that only a subset of the total brown adipocyte population is traced with Myf5-Cre. 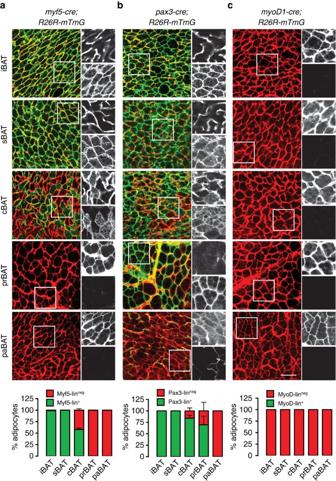Figure 3: The Myf5-Cre and Pax3-Cre lineages are heterogeneously distributed in BAT. (a) Representative images of whole-mount preparations of the indicated BATs of 6-week-oldmyf5-cre;R26R-mTmGmale mice. The mTFP and mGFP channels within the boxed inset are shown enlarged to the right of each panel (top=mTFP; bottom=mGFP). The number of mTFP+and mGFP+mature brown adipocytes in each depot is indicated in a graph at the bottom of each column (n=3–8 mice; mean+s.e.m.). (b) Same asaexcept usingpax3-cre;R26R-mTmGmale mice. (n=3–8; mean+s.e.m.). (c) Same asaandbexcept usingmyod1-cre;R26R-mTmGmale mice. (n=3–4; mean+s.e.m.). Scale bar, 50 μm. Figure 3: The Myf5-Cre and Pax3-Cre lineages are heterogeneously distributed in BAT. ( a ) Representative images of whole-mount preparations of the indicated BATs of 6-week-old myf5-cre;R26R-mTmG male mice. The mTFP and mGFP channels within the boxed inset are shown enlarged to the right of each panel (top=mTFP; bottom=mGFP). The number of mTFP + and mGFP + mature brown adipocytes in each depot is indicated in a graph at the bottom of each column ( n =3–8 mice; mean+s.e.m.). ( b ) Same as a except using pax3-cre;R26R-mTmG male mice. ( n =3–8; mean+s.e.m.). ( c ) Same as a and b except using myod1-cre;R26R-mTmG male mice. ( n =3–4; mean+s.e.m.). Scale bar, 50 μm. Full size image We also find that Pax3-Cre traces a similar population of brown adipocytes. For example, the Pax3-Cre trace mirrors the Myf5-Cre lineage-tracing pattern in iBAT (100% and 99% Pax3-lin + in males and females, respectively) and sBAT (100% in both genders) ( Fig. 3b ; Supplementary Fig. 3b ). However, the Pax3 lineage contributes more than the Myf5 lineage to brown adipocytes in cBAT (84% in males; 91% in females), peri-renal BAT (68% in males; 52% in females) and female paBAT (73%) ( Fig. 3b ; Supplementary Fig. 3b ). We were unable to detect any Pax3-lin + brown adipocytes in male paBAT ( Fig. 3b ). On the other hand, MyoD1-Cre did not label any brown adipocytes confirming that brown adipocytes do not typically arise from MyoD1-expressing precursors ( Fig. 3c ). These data argue that the Pax3 lineage largely overlaps with the Myf5 lineage in iBAT and sBAT, but is more broadly represented in the global brown adipocyte population. Most dorsal-anterior adipocytes are Pax3/Myf5-lin + Next, we quantified the number of mature white adipocytes traced with Myf5-Cre. Because the APC pool in the anterior-subcutaneous WAT (asWAT) contains a mixture of Myf5-lin + and Myf5-lin neg precursors ( Fig. 2a ), we speculated that the mature adipocyte population in this depot would also be a heterogeneous mix. Interestingly, however, we find that almost all of the adipocytes in the asWAT are traced with Myf5-Cre ( Fig. 4a ; Supplementary Fig. 5a ) and the only Myf5-lin neg adipocytes detectable lie in the ventral tip of the depot arranged in a gradient pattern such that the extreme ventral tip is completely Myf5-lin neg ( Supplementary Fig. 5c ). Myf5-Cre also traces 97% and 98% of the mature retroperitoneal WAT (rWAT) adipocytes in males and females, respectively ( Fig. 4a ; Supplementary Fig. 5a ). This again is more than we predicted for this depot based on the Myf5-Cre trace of the APC pool ( Fig. 2a ), which indicates a mixture of Myf5-lin + and Myf5-lin neg APCs (roughly 60:40) that can differentiate into adipocytes in vitro with equal efficiency [8] . In contrast Myf5-Cre does not label any mature pgWAT adipocytes in either sex ( Fig. 4a ; Supplementary Fig. 5a ) consistent with pgWAT APCs being mostly Myf5-lin neg ( Fig. 2a ). Myf5-Cre also does not label any mesenteric WAT (mWAT) adipocytes (we did not examine the mWAT APC pool) ( Fig. 4a ; Supplementary Fig. 5a ) or posterior-subcutaneous WAT (psWAT) adipocytes ( Fig. 4a ; Supplementary Fig. 5a ), which is consistent with most psWAT APCs being Myf5-lin neg ( Fig. 2a ). These data indicate that most of the mature white adipocytes in the dorsal-anterior fat depots in 6-week-old mice are derived from Myf5-lin + precursors. 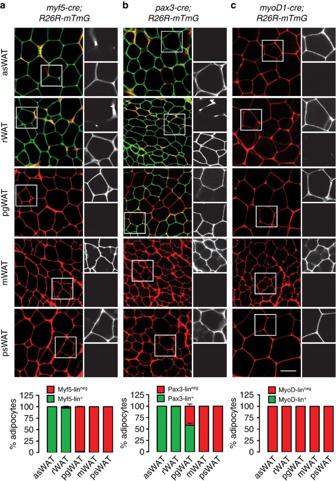Figure 4: Most dorsal-anterior white adipocytes trace with Myf5-Cre and Pax3-Cre. (a) Representative images of whole-mount preparations of the indicated WATs of 6-week-oldmyf5-cre;R26R-mTmGmale mice. The mTFP and mGFP channels within the boxed inset are shown enlarged to the right of each panel (top=mTFP; bottom=mGFP). The number of mTFP+and mGFP+mature white adipocytes in each depot is indicated in a graph at the bottom of each column (n=3–5 mice; mean+s.e.m.). (b) Same asaexcept usingpax3-cre;R26R-mTmGmale mice (n=3–8 mice; mean+s.e.m.). (c) Same asaandbexcept usingmyod1-cre;R26R-mTmGmale mice (n=4 mice; mean+s.e.m.). Scale bar, 50 μm. Figure 4: Most dorsal-anterior white adipocytes trace with Myf5-Cre and Pax3-Cre. ( a ) Representative images of whole-mount preparations of the indicated WATs of 6-week-old myf5-cre;R26R-mTmG male mice. The mTFP and mGFP channels within the boxed inset are shown enlarged to the right of each panel (top=mTFP; bottom=mGFP). The number of mTFP + and mGFP + mature white adipocytes in each depot is indicated in a graph at the bottom of each column ( n =3–5 mice; mean+s.e.m.). ( b ) Same as a except using pax3-cre;R26R-mTmG male mice ( n =3–8 mice; mean+s.e.m.). ( c ) Same as a and b except using myod1-cre;R26R-mTmG male mice ( n =4 mice; mean+s.e.m.). Scale bar, 50 μm. Full size image Next, we examined the Pax3-lineage contribution to the mature white adipocyte population. We find that the Pax3-Cre trace in WAT largely overlaps with the Myf5-Cre pattern in both male and female asWAT and rWAT ( Fig. 4b ; Supplementary Fig. 5b,d ). Also similar to the Myf5-Cre pattern, no mature adipocytes in mWAT or psWAT trace with Pax3-Cre ( Fig. 4b ; Supplementary Fig. 5b ). However, 58% of the male pgWAT adipocytes trace with Pax3-Cre and they are distributed in a variegated pattern throughout the depot ( Fig. 4b ). This is a sharp divergence from the Myf5-Cre trace, which did not mark any male pgWAT adipocytes ( Fig. 4a ), but is consistent with the Pax3-Cre trace to the male pgWAT APC pool ( Fig. 2b ). No adipocytes in female pgWAT trace with Pax3-Cre ( Supplementary Fig. 5b ) confirming a gender-linked difference in lineage distribution. Notably, the Pax3-lin + male pgWAT adipocytes are smaller than the Pax3-lin neg adipocytes cohabitating the same depot ( Supplementary Fig. 5e ) indicating that lineage heterogeneity correlates with size heterogeneity. MyoD1-Cre does not label any white adipocytes ( Fig. 4c ) further confirming that white adipocytes do not typically arise from MyoD1-expressing precursors. Collectively, these data argue that the Pax3 lineage largely overlaps with the Myf5 lineage in asWAT and rWAT, but exhibits a striking gender-linked difference in male pgWAT only. A comparative summary of the lineage-tracing patterns to both BAT and WAT that are described above is depicted in Fig. 5a (for Myf5-Cre) and Fig. 5b (for Pax3-Cre). 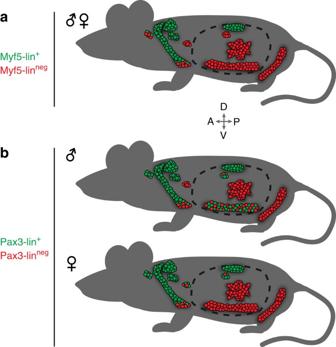Figure 5: Model depicting the Myf5-Cre and Pax3-Cre lineage-tracing patterns. (a) Anatomical distribution of Myf5-Cre-traced adipocytes in BAT and WAT (refer toFig. 1bfor depot identity). The distribution is not significantly different between males and females. Anterior (A), posterior (P), dorsal (D) and ventral (V) are indicated. (b) Anatomical distribution of Pax3-Cre-traced adipocytes in BAT and WAT. Male and female distribution patterns are shown separately because of the gender-linked variation in paBAT and pgWAT. Figure 5: Model depicting the Myf5-Cre and Pax3-Cre lineage-tracing patterns. ( a ) Anatomical distribution of Myf5-Cre-traced adipocytes in BAT and WAT (refer to Fig. 1b for depot identity). The distribution is not significantly different between males and females. Anterior (A), posterior (P), dorsal (D) and ventral (V) are indicated. ( b ) Anatomical distribution of Pax3-Cre-traced adipocytes in BAT and WAT. Male and female distribution patterns are shown separately because of the gender-linked variation in paBAT and pgWAT. Full size image Myf5-lineage distribution is dynamic Next, we wondered whether age or diet influence adipocyte lineage distribution. Interestingly, we find that Myf5-lin neg adipocytes appear in the rWAT of myf5-cre;mTmG mice with age, increasing in prevalence from 0% at 1 week to around 3% at 6 weeks and up to 44% at 6 months ( Fig. 6a ). In contrast, age has no influence on the Pax3-lineage distribution in rWAT, which remains almost exclusively mGFP + at 6 months ( Fig. 6a ). Short-term high-fat diet (HFD; 2 weeks, 45% calories from fat) has similar effects, increasing the percentage of Myf5-lin neg adipocytes in rWAT to around 40% although these mice are young (6 weeks) at the time of analysis ( Fig. 6b ). HFD (similar to age) has no effect on the Pax3-lineage distribution ( Fig. 6b ). Importantly, aging and HFD does not significantly alter the Pax3- or Myf5-lineage contribution to the APC pools in any depot we examined ( Fig. 6c,d ) indicating that the change in Myf5-lineage distribution in the mature adipocyte population is not due to a change in the lineage composition of the precursor pool. We do not observe any differences in the lineage composition of brown fat with age or HFD ( Fig. 6c,d and not shown). In summary, the Myf5-lineage distribution in fat changes in response to both non-modifiable (for example, age) and modifiable (for example, diet) factors while the Pax3-lineage distribution appears to be more static. 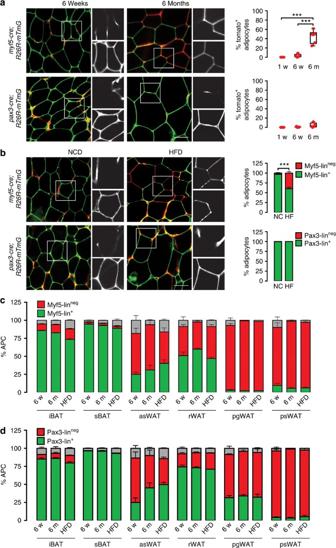Figure 6: The Myf5-Cre-lineage distribution is dynamic. (a) Representative images of whole-mount rWAT frommyf5-cre;R26R-mTmGandpax3-cre;R26R-mTmGmales at 6 weeks and 6 months of age. Quantification of mTFP+(Myf5-Linneg) adipocytes at 1 week, 6 weeks and 6 months of age is shown at the right. Each dot represents one mouse (n=3–6; mean+s.e.m.; ***P<0.001; analysis of variance test). (b) Four-week-oldmyf5-cre;R26R-mTmGandpax3-cre;R26R-mTmGmales were fed a HFD (45% of calories from fat) for 2 weeks and whole-mount preparations of rWAT were imaged at 6 weeks of age. Bar graphs (right) are the quantifications of mTFP+and mGFP+mature rWAT adipocytes in mice fed the normal chow diet (NC) or high-fat diet (HF) (n=5–10 mice formyf5-cre;n=3–8 mice forpax3-cre. mean+s.e.m.; ***P<0.001;t-test). (c) Number of mTFP+and mGFP+APCs isolated from each of the indicated depots frommyf5-cre;R26R-mTmGat 6 weeks of age (6w), 6 months of age (6 m) and from 6 weeks of age after 2 weeks high-fat diet (HFD). A small number of cells in each case that could not be distinguished are indicated in grey (n=3–4; mean+s.e.m.). (d) Same ascexcept usingpax3-cre;R26R-mTmGmice (n=3–6; mean+s.e.m.). Scale bar, 50 μm. Figure 6: The Myf5-Cre-lineage distribution is dynamic. ( a ) Representative images of whole-mount rWAT from myf5-cre;R26R-mTmG and pax3-cre;R26R-mTmG males at 6 weeks and 6 months of age. Quantification of mTFP + (Myf5-Lin neg ) adipocytes at 1 week, 6 weeks and 6 months of age is shown at the right. Each dot represents one mouse ( n =3–6; mean+s.e.m. ; *** P <0.001; analysis of variance test). ( b ) Four-week-old myf5-cre;R26R-mTmG and pax3-cre;R26R-mTmG males were fed a HFD (45% of calories from fat) for 2 weeks and whole-mount preparations of rWAT were imaged at 6 weeks of age. Bar graphs (right) are the quantifications of mTFP + and mGFP + mature rWAT adipocytes in mice fed the normal chow diet (NC) or high-fat diet (HF) ( n =5–10 mice for myf5-cre ; n =3–8 mice for pax3-cre . mean+s.e.m. ; *** P <0.001; t -test). ( c ) Number of mTFP + and mGFP + APCs isolated from each of the indicated depots from myf5-cre;R26R-mTmG at 6 weeks of age (6w), 6 months of age (6 m) and from 6 weeks of age after 2 weeks high-fat diet (HFD). A small number of cells in each case that could not be distinguished are indicated in grey ( n =3–4; mean+s.e.m.). ( d ) Same as c except using pax3-cre;R26R-mTmG mice ( n =3–6; mean+s.e.m.). Scale bar, 50 μm. Full size image Depot differences in brite adipocyte origins Chronic cold temperature or treatment with a β3-adrenergic receptor agonist such as CL316,243 increases the abundance of Ucp1 + multilocular adipocytes in white fat that are called brite (brown in white) adipocytes [16] . We previously proposed that brite adipocytes are derived from both Myf5-lin + or Myf5-lin neg precursors depending upon the depot [8] . To confirm this, we treated myf5-cre;mTmG mice with CL316,243 and asked whether any multilocular adipocytes are mGFP + . We find that all multilocular adipocytes induced by CL316,243 appearing in the asWAT are mGFP + while all multilocular adipocytes appearing in the psWAT are mTFP + ( Fig. 7a ). Interestingly, CL316,243 also induces the formation of nascent mTFP + adipocytes in rWAT, which represent around 40% of the total adipocytes after 1 week of treatment ( Fig. 7b ), thereby changing the Myf5-lineage composition of rWAT in a manner similar to the effects of aging and HFD. As with age and HFD, CL316,243 does not alter the distribution of Myf5-lin + APCs in any depot [7] . This supports the notion that some Myf5-lin + adipocytes may transform into brite adipocytes while others may arise de novo from Myf5-lin neg precursors [3] , [8] , [17] , [18] . To verify that the multilocular adipocytes induced by CL316,243 are indeed brite adipocytes, we analysed whether they express UCP1. By immunohistochemistry, we find that all multilocular cells induced by CL316,243 in psWAT and rWAT strongly stain positive with a UCP1 antibody ( Supplementary Fig. 6a ) consistent with the increase in ucp1 messenger RNA ( Supplementary Fig. 6b ) and protein expression ( Supplementary Fig. 4b ) in these depots after CL316,243 treatment. This suggests that brite adipocytes can be Myf5-lin + or Myf5-lin neg depending upon the depot. 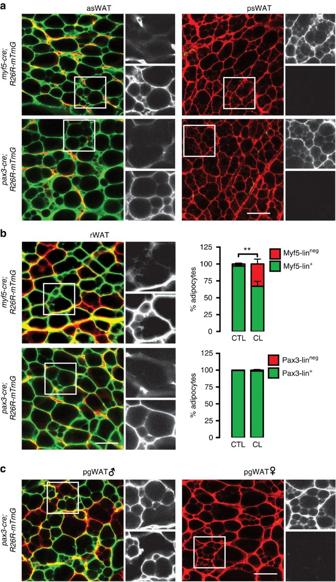Figure 7: Brite adipocytes are Myf5/Pax3-Cre-lineage-positive or -negative depending upon the depot. (a) Representative images of whole-mount preparations of asWAT and psWAT of 6-week-old malemyf5-cre;R26R-mTmG(top) andpax3-cre;R26R-mTmG(bottom) mice that were treated with CL316,243 for 1 week. (b) Representative images of whole-mount preparations of rWAT from malemyf5-cre;R26R-mTmG(top) andpax3-cre;R26R-mTmG(bottom) mice treated with CL316,243 for 1 week starting at 5 weeks of age. (Right) quantification of mTFP+and mGFP+mature adipocytes in the rWAT of control (CTL) and treated (CL) mice is shown (n=4–5 mice formyf5-cre;n=4–8 mice forpax3-cre. mean+s.e.m.; **P<0.01;t-test). (c) Representative images of whole-mount preparations of male and female pgWAT of 6-week-oldpax3-cre;R26R-mTmGmice that were treated with CL316,243 for 1 week. Scale bar, 50 μm. Figure 7: Brite adipocytes are Myf5/Pax3-Cre-lineage-positive or -negative depending upon the depot. ( a ) Representative images of whole-mount preparations of asWAT and psWAT of 6-week-old male myf5-cre;R26R-mTmG (top) and pax3-cre;R26R-mTmG (bottom) mice that were treated with CL316,243 for 1 week. ( b ) Representative images of whole-mount preparations of rWAT from male myf5-cre;R26R-mTmG (top) and pax3-cre;R26R-mTmG (bottom) mice treated with CL316,243 for 1 week starting at 5 weeks of age. (Right) quantification of mTFP + and mGFP + mature adipocytes in the rWAT of control (CTL) and treated (CL) mice is shown ( n =4–5 mice for myf5-cre ; n =4–8 mice for pax3-cre . mean+s.e.m. ; ** P <0.01; t -test). ( c ) Representative images of whole-mount preparations of male and female pgWAT of 6-week-old pax3-cre;R26R-mTmG mice that were treated with CL316,243 for 1 week. Scale bar, 50 μm. Full size image We next asked whether CL316,243 induces Pax3-lin + brite adipocytes in the pax3-cre;mTmG mice. Similar to the case with the Myf5 lineage nearly all of the multilocular adipocytes induced by CL316,243 in the asWAT and rWAT are mGFP + ( Fig. 7a ). However, unlike in the myf5-cre;mTmG mice, no nascent mTFP + brite adipocytes are detectable in the rWAT following CL316,243 treatment ( Fig. 7b ) further suggesting that the Pax3 lineage is more static. In male pgWAT, CL316,243 also induces the formation of both mGFP + and mTFP + brite adipocytes without affecting Pax3-lineage distribution ( Fig. 7c ). CL316,243 also does not affect the Pax3-lineage distribution in any APC population examined ( Supplementary Fig. 6c,d ). In sum, these data obtained from a survey of all major depots argue that although most brite adipocytes reside in the psWAT, these cells cannot be generally classified as being Myf5-lineage-positive or -negative (or Pax3-lineage-positive or -negative) because brite adipocytes residing in other depots can also be traced with Myf5-Cre or Pax3-Cre. Adipocyte lineages have plasticity We previously discovered that deleting PTEN (a negative regulator of insulin/PI3K signalling) with Myf5-Cre results in a body fat distribution phenotype in which iBAT, sBAT, asWAT and rWAT (the Myf5-lin + depots) expand while the psWAT, mWAT and pgWAT (the Myf5-lin neg depots) disappear [8] . Furthermore, by lineage tracing with the R26R-YFP reporter we found that deleting PTEN with Myf5-Cre selectively expands the Myf5-lin + APC population at the expense of Myf5-lin neg APCs. We therefore predicted that all mature adipocytes in these mice are likely Myf5-lin + . To test this, we generated PTEN myf5cKO mice that additionally carry the R26R-mTmG reporter ( myf5-cre;PTEN fl/fl ;mTmG ). Lineage tracing with the R26R-mTmG reporter confirms that there is an expansion of the Myf5-lin + APCs in the PTEN myf5cKO mice ( Supplementary Fig. 7a ) and that all mature adipocytes in these mice are indeed traced with Myf5-Cre ( Supplementary Fig. 7b ). Thus, differences in insulin/PI3K signalling between lineages can alter the lineage composition of adipose tissue. To further investigate the role of insulin signalling in Myf5-lineage adipocytes, we generated myf5-cre;IR β fl/fl conditional knockout ( IR myf5cKO ) mice. Six-week-old IR myf5cKO mice show no significant difference in total body weight compared with controls ( Fig. 8a ) and no overall difference in individual lean tissue mass ( Supplementary Fig. 8a ). However, iBAT, sBAT, cBAT and rWAT weigh over threefold less in the IR myf5cKO mice ( Fig. 8b,c ) while the mass of psWAT and pgWAT is increased ( Fig. 8c ). Despite altered fat distribution, the IR myf5cKO mice have normal insulin, glucose and cold tolerance ( Supplementary Fig. 8b–d ). Thus, IR myf5cKO mice have a body fat distribution phenotype characteristically opposite to the PTEN myf5cKO mice. 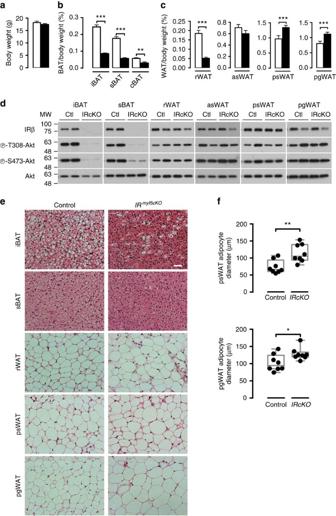Figure 8:IRmyf5cKOmice have altered body fat distribution. (a) Total body weight ofIRmyf5cKOand littermate control mice at 6 weeks of age (n=14 mice). (b) BAT mass relative to body weight for the indicated depots at 6 weeks of age (n=14 mice; mean+s.e.m.; **P<0.01; ***P<0.001;t-test). (c) WAT mass relative to body weight for the indicated depots at 6 weeks of age (n=14 mice; mean+s.e.m.; ***P<0.001;t-test). (d) Western blots of the indicated tissues fromIRmyf5cKOand littermate control mice at 6 weeks of age. (e) Haematoxylin and eosin images of the indicated BATs and WATs fromIRmyf5cKOand control mice at 6 weeks of age. (f) Cell size quantification of mature adipocytes from psWAT and pgWAT ofIRmyf5cKOand littermate control mice at 6 weeks of age (n=8 mice; boxplot indicating maximum, minimum, media and all data points; *P<0.05; **P<0.01;t-test). Figure 8: IR myf5cKO mice have altered body fat distribution. ( a ) Total body weight of IR myf5cKO and littermate control mice at 6 weeks of age ( n =14 mice). ( b ) BAT mass relative to body weight for the indicated depots at 6 weeks of age ( n =14 mice; mean+s.e.m. ; ** P <0.01; *** P <0.001; t -test). ( c ) WAT mass relative to body weight for the indicated depots at 6 weeks of age ( n =14 mice; mean+s.e.m. ; *** P <0.001; t -test). ( d ) Western blots of the indicated tissues from IR myf5cKO and littermate control mice at 6 weeks of age. ( e ) Haematoxylin and eosin images of the indicated BATs and WATs from IR myf5cKO and control mice at 6 weeks of age. ( f ) Cell size quantification of mature adipocytes from psWAT and pgWAT of IR myf5cKO and littermate control mice at 6 weeks of age ( n =8 mice; boxplot indicating maximum, minimum, media and all data points; * P <0.05; ** P <0.01; t -test). Full size image Consistent with our lineage-tracing experiments, IRβ levels and AKT phosphorylation are reduced in the IR myf5cKO iBAT and sBAT ( Fig. 8d ). Also consistent, IRβ levels and AKT phosphorylation are normal in the Myf5-lin neg psWAT and pgWAT ( Fig. 8d ). In contrast to our lineage-tracing results, IRβ levels and AKT phosphorylation are also similar to controls in the rWAT and asWAT ( Fig. 8d ). This was unexpected because most of the mature adipocytes in these depots trace with Myf5-Cre. Histological analysis indicates that most of the IRβ-deficient brown adipocytes are smaller because they have reduced lipid content ( Fig. 8e ) consistent with a role for insulin in driving lipogenesis genes in BAT including srebp1c (sterol regulatory-binding protein 1c), acl (ATP-citrate lyase), acc (acetyl-CoA carboxilase) and fas (fatty acid synthase) ( Supplementary Fig. 8e ). Notably, however, a few interspersed brown adipocytes containing normal lipid droplet content are detectable in the mutant BATs ( Fig. 8e ), suggesting that a small number of brown adipocytes might also be IRβ-positive. The adipocytes in the IR myf5cKO rWAT, asWAT, psWAT and pgWAT exhibit the typical white adipocyte appearance of having a single large lipid droplet ( Fig. 8e and not shown). Cell size analysis also reveals that the mature adipocytes in the psWAT and pgWAT of the IR myf5cKO mice are larger (hypertrophic) than the corresponding adipocytes in controls ( Fig. 8e,f ) likely explaining at least in part why these depots weigh more in the mutant. Why are IRβ levels normal in the rWAT and asWAT of IR myf5cKO mice when these depots are normally traced with Myf5-Cre? We hypothesized that the apparent contradiction could reflect lineage plasticity. To test this, we generated myf5-cre;IR β fl/fl ;mTmG mice to ask whether Myf5-lin neg (mTFP + ) adipocytes replace Myf5-lin + (mGFP + ) adipocytes in the mutant rWAT and asWAT. This is indeed the case; while deleting IR β with Myf5-cre does not significantly affect the Myf5-lineage composition of the APC pool in either depot ( Fig. 9a ) it completely changes the lineage composition of the mature adipocyte population ( Fig. 9b ). For example, the mature adipocytes in the mutant asWAT and rWAT, which are normally Myf5-lin + , are entirely Myf5-lin neg in the IR myf5cKO mice ( Fig. 9b ). Notably, the Myf5-lin + (mGFP + ) IRβ knockout cells are detectable in the mutant rWAT and asWAT, but they are much smaller and interspersed among the larger lipid-filled Myf5-lin neg adipocytes ( Fig. 9b ). Thus, IRβ is not essential in the Myf5 lineage for establishing APCs but it is essential for adipogenesis. 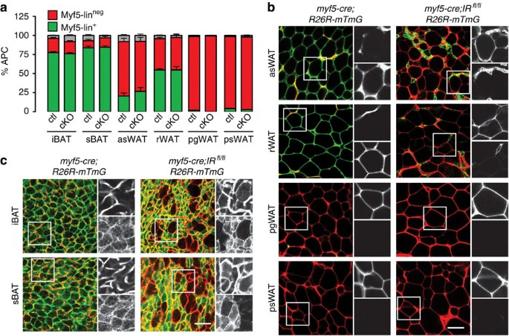Figure 9: Adipocyte lineages have plasticity. (a) Number of mTFP+and mGFP+APCs isolated from each of the indicated depots from 6-week-old maleIRmyf5cKO-R26R-mTmGand control mice (n=10 males; mean+s.e.m.). (b,c) Representative images of whole-mount preparations of the indicated WATs (b) and BATs (c) of 6-week-oldIRmyf5cKO-R26R-mTmGmice. Scale bar, 50 μm. Figure 9: Adipocyte lineages have plasticity. ( a ) Number of mTFP + and mGFP + APCs isolated from each of the indicated depots from 6-week-old male IR myf5cKO -R26R-mTmG and control mice ( n =10 males; mean+s.e.m.). ( b , c ) Representative images of whole-mount preparations of the indicated WATs ( b ) and BATs ( c ) of 6-week-old IR myf5cKO -R26R-mTmG mice. Scale bar, 50 μm. Full size image In the mutant iBAT and sBAT, the more abundant smaller brown adipocytes are all mGFP + consistent with the robust decrease in IRβ and phospho-AKT levels in these depots ( Fig. 8d ). However, the few large adipocytes detectable in these depots are Myf5-lin neg (mTFP + ) ( Fig. 9c ) indicating that some expansion of Myf5-lin neg (IRβ + ) brown adipocytes also occurs in IR myf5cKO mice. However, there is no compensatory ‘browning’ in psWAT (that is, increased multilocularity and ucp1 induction) as would be expected if BAT were completely dysfunctional ( Fig. 8e ; Supplementary Fig. 8f ) [19] . Collectively, these findings indicate that adipocyte lineages have plasticity. In this study, we compare the lineage-tracing patterns of Myf5-Cre, Pax3-Cre and MyoD1-Cre in adipose tissue using a reporter optimal for labelling mature adipocytes. We provide evidence that only a subset of brown adipocytes arise from Myf5-Cre-expressing precursors. Furthermore, we find that most dorsal-anterior white adipocytes also derive from Myf5-Cre-expressing precursors, and that there is a large degree of overlap between the Pax3-Cre and Myf5-Cre lineages in both brown and white adipocytes. In contrast, no adipocytes trace to MyoD1-Cre-expressing precursors. Finally, we find that adipocyte lineages are not necessarily fixed, but can vary with gender, and in response to modifiable and non-modifiable factors. On the basis of these findings, we propose a revised model of the Myf5-lineage contribution to adipose tissue ( Fig. 10 ) and the following concepts in adipose tissue development: first, adipocytes originate from multiple developmental lineages that are distributed heterogeneously in depot-specific patterns; second, adipocyte lineage contribution to the mature adipocyte pool varies with age; third, adipocyte lineages may selectively expand in response to certain factors; fourth, adipocyte lineages can compensate for each other indicating that lineage plasticity exists. Another study found that cephalic adipocytes arise from neural crest precursors further supporting the model in which adipocytes have multiple developmental origins [20] . Although we do not yet know the origin of the Pax3/Myf5-lineage-negative adipocytes in our study, we hypothesize that they may arise from multiple distinct lineages that might be dynamically distributed in patterns similar to those described here. Thus, our work provides a conceptual framework for future investigations. 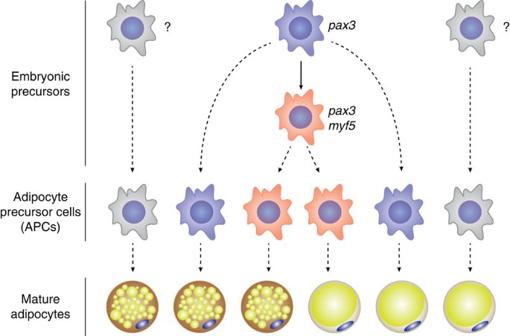Figure 10: A revised model of adipocyte origins based on Pax3-Cre and Myf5-Cre lineage tracing to mature adipocytes. Embryonic precursors expressing Pax3-Cre and Myf5-Cre give rise to a subset of APCs and mature brown and white adipocytes. A subset of brown and white adipocytes also arises from Pax3-Cre+precursors that do not express Myf5-Cre. The origin of Pax3-Cre- and Myf5-Cre-negative adipocytes is not yet clear. Dotted lines are used to indicate lineages because the intermediate stages are poorly understood. Note that the knockin Cre drivers used in this study are indicative of the activity of the endogenous promoters. Figure 10: A revised model of adipocyte origins based on Pax3-Cre and Myf5-Cre lineage tracing to mature adipocytes. Embryonic precursors expressing Pax3-Cre and Myf5-Cre give rise to a subset of APCs and mature brown and white adipocytes. A subset of brown and white adipocytes also arises from Pax3-Cre + precursors that do not express Myf5-Cre. The origin of Pax3-Cre- and Myf5-Cre-negative adipocytes is not yet clear. Dotted lines are used to indicate lineages because the intermediate stages are poorly understood. Note that the knockin Cre drivers used in this study are indicative of the activity of the endogenous promoters. Full size image Using the same Myf5-Cre knockin allele employed in this study, a previous study concluded that Myf5 + precursors give rise to all brown adipocytes and myocytes, but not to any white adipocyte [10] . Why Seale et al . [10] arrived at a different conclusion is unclear but could reflect the use of a lineage-tracing reporter that is suboptimal for labelling mature adipocytes or limiting the analysis to a few depots. Seale et al . [10] also concluded that all brite adipocytes (sometimes called beige adipocytes) arise from a Myf5 neg lineage. However, our results suggest that brite adipocytes can descend from precursors that are either Myf5-Cre (or Pax3-Cre)-positive or -negative depending upon the depot. Most studies of brite/beige adipocytes focus on psWAT likely explaining why this was previously missed. Notably, the Cre drivers used in this study are knockin alleles meaning that Cre expression reflects the activity of the endogenous promoter. While this is ideal for lineage tracing, whether Myf5 and Pax3 proteins co-express or have a functional role in adipocyte development cannot be inferred from studies using these drivers. It also cannot be determined whether the Myf5-Cre and Pax3-Cre drivers express in precursor cells that are common to both myocytes and adipocytes or in separate co-existing lineages. Nevertheless, our results favour a model in which brown and white adipocytes have multiple developmental origins, a subset of which can be defined by Myf5 and/or Pax3 promoter expression. The in vivo regulation of adipose tissue development is poorly understood in part because, without knowing the developmental origins of adipocytes, tools to genetically target adipocyte lineages have been lacking. Previous in vivo genetic studies of adipocyte regulation have largely relied on Cre drivers that express in mature adipocytes [21] , [22] . Taking advantage of the fact that Myf5-Cre targets precursors to both brown and white adipocytes, we investigated the function of the insulin receptor in adipocyte development. Consistent with the hypothesis that preadipocytes become insulin dependent during differentiation [23] , we found that IRβ is required in the Myf5 lineage for adipogenesis but not for establishing APCs, and that Myf5-lin neg adipocytes can increase in abundance and size to compensate. Such plasticity has been reported previously in skeletal muscle in which Myf5 and MyoD define different skeletal muscle lineages that can compensate for each other during development [24] , [25] . However, we also observed that while adipocyte lineages have plasticity, the degree of plasticity varies depending upon the depot. For example, while Myf5-lin neg adipocytes fully compensate for IR β knockout lineages in asWAT (indicated by the normal size of this depot in the IR myf5cKO mice), the rWAT is much smaller in the mutant suggesting Myf5-lin neg adipocytes can only partially compensate in this depot. Notably, the degree to which Myf5-lin neg adipocytes compensate is roughly proportional to the number of Myf5-lin neg APCs present in each depot ( Fig. 2a ). Despite this depot-dependent variation in lineage plasticity, however, the IR myf5cKO mice maintain similar total body mass as controls by additionally increasing the mass (by increasing individual cell size) of the psWAT and pgWAT depots. This combined presence of lipoatrophy and lipohypertrophy is often observed in human partial lipodystrophy syndromes [5] . While lineage tracing in mammals currently can only be performed in mice, we hypothesize that the concepts outlined here may help explain in humans some of the heterogeneity observed within and between adipose tissue depots, body fat patterning variations in the population and/or the pathology of certain lipodystrophies. Further elucidating other developmental origins of adipocytes, the signals regulating their distribution and their functional differences will be critical to understanding the pathogenesis of obesity and obesity-associated complications. Materials Antibodies to IRβ, P-T308-Akt, P-S473-Akt and Pan-Akt (all used at 1/1,000 dilution) were from Cell Signaling. UCP1 antibody (#10983) was from AbCam (used at 1/100 for IHC and at 1/1,000 for western blot). Live/dead Blue (Molecular Probes, L23105), CD31-PE-CY7 (eBioscience, 25-0311)(used at 1/1,000), CD45-PE-CY7 (eBioscience, 25-0451) (used at 1/1,000), CD29-AlexaFluor700 (Biolegend, 102218)(used at 1/400), CD34-AlexaFluor647 (Biolegend, 119314)(used at 1/200), Sca1-Pacific Blue (BD Bioscience, 560653)(used at 1/1,000) and CD45-FITC (eBioscience, 11-0451) (used at 1/200) were used for flow cytometry. CL316,243 was from Tocris. Mice myf5-cre (stock 007893), R26R-mTmG (stock 007676), pax3-cre (stock 005549), myoD1-cre (stock 01440), adiponectin-cre (stock 010803) and IRβ (stock 006955) mice were from Jackson Laboratory. Mice were housed in the Animal Medicine facilities of the UMMS in a room set at 22 °C and 45% humidity under daily 12 h light/dark cycles. All animal experiments were approved by the University of Massachusetts Medical School animal care and use committee. In vivo experiments For high-fat diet experiments, 4-week-old male and female mice were fed a high-fat diet of 45% calories from fat (Research Diets) for 2 weeks. CL316,243 (1 mg kg −1 of body weight) and vehicle control were administered in phosphate-buffered saline via intraperitoneally (i.p.) in 5-week-old male and female mice for 1 week. Both, high-fat diet and CL316,243-treated mice were analysed at 6 weeks of age. Overnight 6-week-old fasted male and females were subjected to glucose tolerance test by injecting glucose at 2 g kg −1 of body weight by i.p. injection. Insulin tolerance tests were performed in 6-h fasted animals. Insulin (HumulinR) was administrated at 0.75 U kg −1 of body weight by i.p. injection. Blood glucose was measured by tail bleeding using a commercial blood glucose tester. For acute cold challenge 6-week-old males and female mice were transferred to pre-acclimated cages in a cold room and rectal temperature was measured every hour using the Microtherma 2 system (Braintree Scientific Inc.). Gene expression and western blot Total RNA was isolated from cells or tissues using Qiazol (Invitrogen) and an RNeasy kit (Invitrogen). Equal amounts of RNA were retro-transcribed to complementary DNA using a High Capacity cDNA reverse transcription kit (#4368813, Applied Biosystems). Quantitative reverse transcriptase-PCR was run in 10-μl reactions in a StepOnePlus real-time PCR machine from Applied Biosystems using SYBR Green PCR master mix (#4309156, Applied Biosystems) according to the manufacturer’s instructions. Standard and melting curves were run in every plate for every gene to ensure efficiency and specificity of the reaction. Primer sequences: TBP Fw: 5′-GAAGCTGCGGTACAATTCCAG-3′, TBP Rv: 5′-CCCCTTGTACCCTTCACCAAT-3′, SREBP1c Fw: 5′-AAGCAAATCACTGAAGGACCTGG-3′, SREBP1c Rv: 5′-AAAGACAAGCTACTCTGGGAG-3′, ACL Fw: 5′-CTCACACGGAAGCTCCATAA-3′, ACL Rv: 5′-ACGCCCTCATAGACACCATC-3′, ACC Fw: 5′-GGAGATGTACGCTGACCGAGAA-3′, ACC Rv: 5′-ACCCGACGCATGGTTTTCA-3′, FAS Fw: 5′-GCTGCGGAAACTTCAGGAAAT-3′, FAS Rv: 5′-AGAGACGTGTCACTCCTGGACTT-3′, UCP1 Fw: 5′-CTGCCAGGACAGTACCCAAG-3′, UCP1 Rv: 5′-TCAGCTGTTCAAAGCACACA-3′, PRDM16 Fw: 5′-GACATTCCAATCCCACCAGA-3′, PRDM16 Rv: 5′-CACCTCTGTATCCGTCAGCA-3′, cidea Fw: 5′-ATCACAACTGGCCTGGTTACG-3′, cidea Rv: 5′-TACTACCCGGTGTCCATTTCT-3′, tdTomato Fw: 5′-GCTGAAGGGCGAGATCCA-3′, tdTomato Rv: 5′-GTGGGAGGTGATGTCCAGCTT-3′, eGFP Fw: 5′-CATGCCCGACTACGT-3′, eGFP Rv: 5′-GCTTGTGCCCCAGGATGTT-3′. For western blot, tissues were homogenized using a TissueLyser (Qiagen) system in a buffer containing 50 mM Hepes, pH 7.4, 40 mM NaCl, 2 mM EDTA, 1.5 mM NaVO 4 , 50 mM NaF, 10 mM sodium pyrophosphate, 10 mM sodium β-glycerophosphate, 0.1% SDS, 1% sodium deoxycholate and 1% Triton X-100. An equal amount of total protein was loaded into acrylamide/bis-acrylamide gels and transferred to PVDF membranes for detection with the indicated antibodies. All antibodies for western blot were used at dilution 1/1,000. UCP1 IHC Fat sections were subjected to UCP1 IHC according to ref. 26 . Briefly, fat sections were re-hydrated and antigen retrieval was done by incubating the sections in citrate buffer at 90–95 °C water for 20 min. After blocking, primary antibody was applied overnight at 4 °C. The next day, SuperPicture 3 rd Gen IHC Detection Kit (Novex) was used for detection. Tissue harvest Adipose tissues used were carefully dissected to avoid surrounding tissue contamination. Adipose tissue notation used here was described previously [8] , [27] . psWAT is equivalent to inguinal WAT and paBAT is equivalent to mediastinic BAT in ref. 27 . APC isolation and FACS analysis APCs were isolated as follows [8] , [28] : stromal-vascular fraction was prepared from each fat pad by collagenase treatment and stromal-vascular fraction pellets were resuspended in erythrocyte lyses buffer (0.15 M ClNH 4 and 0.01 M HCO 3 K in water). Cells were then pelleted by centrifugation, resuspended in staining media (Hanks’ balanced salt solution+2% fetal bovine serum) and labelled with appropriate antibodies. After staining, cells were filtered through a 35-μm cell-strainer capped tube to ensure single-cell suspension and stained with live/dead Blue. Live single cells were gated according to the expression of surface markers (CD31 − CD45 − CD29 + CD34 + Sca1 + ) in a BD LSRII analyser. Data were analysed with FlowJo. Whole-mount confocal microscopy Fats were dissected and cut in ~5 × 5 mm cubes. Fragments were mounted with Fluoromount-G (Southern Biotech). Mounted samples were imaged the same day on a LSM 5 Pascal (Zeiss) point scanner confocal system. To acquire the images for quantification, a general survey of the entire tissue was first performed using a × 10 objective to determine the uniformity of labelling throughout the tissue. Then, the tissue was subdivided into quadrants and a × 40 oil immersion objective was used to obtain random images from each quadrant. Background fluorescence was offset using tissues from animals not carrying the R26R-mTmG reporter. tdTomato and enhanced green fluorescent protein (eGFP) settings were set using fat tissues from mice carrying the R26R-mTmG reporter and from adiponectin-Cre;R26R-mTmG mice, respectively. eGFP was excited at 488 nm and detected from 515 to 565 nm. tdTomato was excited at 543 nm and detected from 575 to 640 nm. Histology and image analysis For muscle histology, fresh dissected muscles were flash-frozen in optimal cutting temperature compound (OCT) using dry-ice cold isopentane. Frozen transversal sections (10 μm) were obtained and mounted in Prolong Gold. Images were taken on the same day on a LSM 5 Pascal (Zeiss) point scanner confocal system. ImageJ (NIH) was used to calculate adipocyte diameter in formalin-fixed tissues that were sectioned at 5 μm thickness. Embedding and sectioning was done by the UMass Morphology Core. ImajeJ was used for tdTomato and eGFP channel isolation. Cell counter plug-in of ImageJ was used to count by hand the tdTomato/eGFP adipocytes. More than 100 adipocytes per tissue were counted. Statistical analysis Data are presented as mean+s.e.m., unless stated otherwise. Student’s t -test or analysis of variance, as appropriate, were used to determine statistical significance ( P <0.05). No pre-test was used to choose sample size. No data points were excluded. Statistical analysis was done using GraphPad Prism v6.0c. The number of mice used per experiment is stated in each figure legend. How to cite this article: Sanchez-Gurmaches, J. & Guertin, D. A. Adipocytes arise from multiple lineages that are heterogeneously and dynamically distributed. Nat. Commun. 5:4099 doi: 10.1038/ncomms5099 (2014).